Chalcogen bond-guided conformational isomerization enables catalytic dynamic kinetic resolution of sulfoxides Conformational isomerization can be guided by weak interactions such as chalcogen bonding (ChB) interactions. Here we report a catalytic strategy for asymmetric access to chiral sulfoxides by employing conformational isomerization and chalcogen bonding interactions. The reaction involves a sulfoxide bearing two aldehyde moieties as the substrate that, according to structural analysis and DFT calculations, exists as a racemic mixture due to the presence of an intramolecular chalcogen bond. This chalcogen bond formed between aldehyde (oxygen atom) and sulfoxide (sulfur atom), induces a conformational locking effect, thus making the symmetric sulfoxide as a racemate. In the presence of N–heterocyclic carbene (NHC) as catalyst, the aldehyde moiety activated by the chalcogen bond selectively reacts with an alcohol to afford the corresponding chiral sulfoxide products with excellent optical purities. This reaction involves a dynamic kinetic resolution (DKR) process enabled by conformational locking and facile isomerization by chalcogen bonding interactions. Non–covalent interactions based on hydrogen bond [1] , [2] , [3] and halogen bond [4] , [5] , [6] , [7] represent a powerful and promising activation mode in catalytic synthesis. However, the chalcogen bond is a new class of weak non–covalent interactions between the chalcogen atom (S, Se, Te) and Lewis base (Fig. 1a ), which attracted attentions only in recent years [8] , [9] , [10] . In the living systems, the chalcogen bonding interactions play a crucial role in regulating protein conformations [11] and preserving certain enzymatic activities [12] , [13] (Fig. 1b ). These interactions have also been studied in the areas of solid–state chemistry [14] , anion recognition [15] , [16] , [17] , supramolecular assembling [18] , [19] , [20] , and drug designs [21] , [22] . For example, the conformational locking effect induced by chalcogen bonds is believed to enhance the bioactivities of multiple commercial pharmaceuticals such as Acetazolamide [23] and Selenazofurin [24] . (Fig. 1b ). In contrast to the relatively wide applications in functional molecule design, chalcogen bonds are much less explored as effective tools for catalysis and organic synthesis especially in asymmetrical reactions [25] . The use of chalcogen bonding (ChB) for catalysis received reasonable attentions only in recent years [26] , [27] . As disclosed by Matile [28] , [29] , Huber [30] , [31] and Wang [32] , [33] , [34] , the key is to install chalcogen bond donors to the catalysts that can interact with the substrate for catalytic activations (Fig. 1c ). Most of the success for effective catalysis comes from cationic chalcogen bonding interactions, which cationic charges are introduced to decrease the electron density of chalcogen atom to enhance chalcogen bonding interaction. Despite these impressive progresses, the development of effective chalcogen bonding catalysis remains slow, and evidences for the presence of chalcogen bond in catalytic reactions mostly relies on in situ NMR spectra ( 13 C, 77 Se) [27] , [32] , [33] , [34] , [35] , UV-vis and nanoESI-MS [15] analysis. We postulate that part of the reasons lie on the difficulties in designing these stable chalcogen bonded complex between catalysts and substrates. Fig. 1: Chalcogen bonding in functional molecules and asymmetric synthesis. a Chalcogen bond (ChB). b ChB in living systems, medicines, and agrochemicals. c Intermolecular (cationic) ChB in organic catalysis. d Intramolecular (neutral) ChB of substrate as enabling tools for asymmetric synthesis (of chiral sulfoxides). e Examples of functional chiral sulfoxides. Full size image We’re particularly motivated by the fact that such intramolecular interactions are widely present (or can be readily installed) in both macro [18] , [19] , [20] and small molecules of natural origins [11] , [12] , [13] or chemical synthesis [25] , [26] , [27] , [28] , [29] , [30] , [31] , [32] , [33] , [34] , [36] . It is also encouraging to observe that chalcogen bonding in the intramolecular fashion can be designed in readily predictable and modular manners [21] , [22] , [23] , [24] . For instance, Tomada et al reported a chiral selenenylation reagent bearing the intramolecular N-Se interaction to rigidify the whole molecule [37] . Subsequently, Wirth extended this concept towards O-Se interactions and achieved the asymmetric functionalization of alkenes [38] . Furthermore, the transient intramolecular chalcogen bonding interactions had been proven by Smith et al which were the crucial force in stereoselectivity control [25] , [39] , [40] , [41] , [42] , [43] , [44] . Based on these thought-provoking applications of intramolecular ChBs [45] , [46] , [47] , [48] , our interests are directed toward employing intramolecular chalcogen bonding interactions for conformational regulations and selective chemical transformations. In this work, we study the involvement of ChB interactions in the reactivity of sulfinyldibenzaldehyde compounds. These noncovalent interactions are key to achieve the regioselective mono-esterification of the compound via chiral carbene-catalyzed oxidation process, enabling the preparation of chiral sulfoxides. These results indicate that ChB interactions can play an important role in asymmetric organic synthesis. Reaction development Here we disclosed a catalytic dynamic kinetic resolution protocol of sulfoxides which were enabled by intramolecular chalcogen bond–guided conformational isomerization of the substrate (Fig. 1d ). The sulfoxide group have been testified to be a ChB donor [8] , [49] and the solid–state X–ray structure of 1a (Fig. 1d , details see Supplementary Table 2 ) suggests the presence of chalcogen bond between sulfur and oxygen atom (bond length = 2.861 Å). 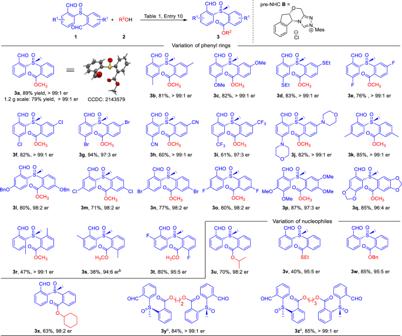Fig. 2: Substrates scope of the reactiona. aReaction conditions as stated in Table1, entry 10. Yields are isolated yields after purification by column chromatography. Er values were determined via HPLC on chiral stationary phase.b50 °C and THF as solvent.c220 mol%1a, DQ, K3PO4and 100 mol% diol were used. This chalcogen bond breaks the symmetry of 1a , and therefore makes this symmetric sulfoxide present as a racemic mixture with two conformational enantiomers [( R p )– 1a and ( S p )– 1a , Fig. 1d ]. Interconversion of the two enantiomers via chalcogen bond–guided conformational isomerization was estimated by DFT, which was a facile process with an activation energy of 8.55 kcal/mol. We postulated that the chalcogen bonding likely exist in solution as well, and then started to screen suitable conditions for a dynamic kinetic resolution of such conformers by using an NHC–catalyzed esterification process. Under the catalysis of N–heterocyclic carbene (NHC) [50] , [51] , [52] , [53] , [54] at an oxidative condition to covert one of the aldehyde moieties of 1a to an ester, a highly efficient dynamic kinetic resolution of this sulfoxide ( 1a ) is realized. Oxidation of Breslow intermediates to the corresponding acyl azolium intermediates ( I and I’ ) were estimated (via DFT) to be the stereoselectivity–determining step in this DKR process. Our reaction affords chiral sulfoxide products with good yields and excellent enantiomeric purities. Notably, chiral sulfoxides are widely used in medicines (such as Esomeprazole [55] and Armodafinil [56] ), agrochemicals (such as Ethiprole [57] ), and as ligands in asymmetric catalysis [58] , [59] (Fig. 1e ). 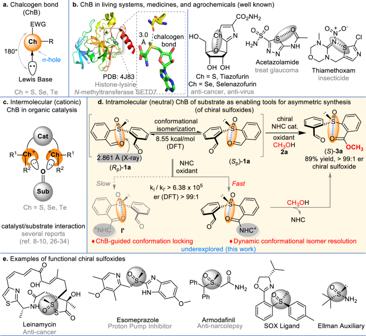The chiral sulfoxides from our reactions may work as platform scaffolds for transforming to bioactive molecules and catalysts. Fig. 1: Chalcogen bonding in functional molecules and asymmetric synthesis. aChalcogen bond (ChB).bChB in living systems, medicines, and agrochemicals.cIntermolecular (cationic) ChB in organic catalysis.dIntramolecular (neutral) ChB of substrate as enabling tools for asymmetric synthesis (of chiral sulfoxides).eExamples of functional chiral sulfoxides. At first, we chose conformational isomeric sulfinyldibenzaldehyde 1a as the model sulfoxide substrate and methanol 2a as a nucleophile to search for suitable conditions, and the key results were summarized in Table 1 . Triazoliums were explored as the NHC pre–catalysts with diphenoquinone (DQ) [60] as an oxidant to convert one of the aldehyde moieties of 1a to an ester unit. An encouraging result was obtained when aminoindanol–derived triazoium A was the NHC pre–catalyst with K 2 CO 3 as a base in THF, offering the corresponding chiral sulfoxide product 3a in 45% yield and 99:1 er (entry 1). Replacing the counter anion (BF 4 − ) in A with a chloride ion (pre–catalyst B ) led to comparable results for this model substrate (entry 2). As an important technical note, in subsequent studies for scope explorations, we found that pre–catalyst B consistently performed better for all the substrate examinations. The N–mesityl substituent in A could be switched by a phenyl unit (pre–catalyst C ) with little effect on product yield or er value (entry 3). Further optimizations with respects to bases and solvents were performed by using NHC pre–catalyst B (entries 5–12). At last, we found that by using K 3 PO 4 as the base with CH 2 Cl 2 as the solvent, product 3a could be isolated in 89% yield with over 99:1 er (entry 10). Table 1 Optimization of reaction conditions a Full size table Substrate scope Having an acceptable condition in hand, the generality of the reaction was then investigated (Fig. 2 ). Various substituents were placed on the para–carbon (relative to the aldehyde moiety) on the phenyl ring of 1a , in all cases the mono–ester products were obtained with excellent er values (mostly over 99:1 er, 3b to 3j ). The reaction yields are good as well when the substituents are methyl ( 3b ), methoxyl ( 3c ), ethylthio ( 3d ) or halogen atoms ( 3e–3g ), giving the corresponding products with 60–94% yields. When electron–withdrawing units (e.g., CN, CF 3 ) were used, the products ( 3 h, 3i ) were obtained in slightly lower yields (60% and 61% yields) with excellent er values maintained. The main side products were from further esterification reaction of 3 h and 3i to give the corresponding di–ester adducts. Various substituents (such as Me, OBn and halogen) could be installed on the meta–carbon (relative to the aldehyde) on the phenyl ring of 1a as well without affecting reaction yields and er values ( 3k–3o ). Remarkably, substrates with two substituents on both the para– and meta–carbons of 1a were well tolerated ( 3p and 3q ). When a methyl unit was placed on the ortho–position (relative to aldehyde) of 1a , drops on both reaction yield and er value were observed ( 3 s ). The low yield of 3 s was mainly due to di–ester formation, and the origins for the decrease of er value may result from steric hindrance. Fluorine substituent at ortho–position led to product 3t with 80% yield and 95:5 er. Placing a methyl unit on the ortho–carbon (relative to the sulfoxide unit) of 1a led to 3r with over 99:1 er, albeit with a decreased 47% yield. Moreover, various alcohols and thiols, including secondary alcohols, could also be used as effective nucleophiles to replace methanol ( 3u–3x ). Interestingly, when diols were used as the nucleophiles, both of hydroxyl moieties could be acylated to give the corresponding chiral di–sulfoxides with excellent yields and er values ( 3 y , 3z ). These results suggested that our strategy may be further developed to attach chiral sulfoxide to functional molecules (such as natural products and polymers) which contain multiple hydroxyl units. Fig. 2: Substrates scope of the reaction a . a Reaction conditions as stated in Table 1 , entry 10. Yields are isolated yields after purification by column chromatography. Er values were determined via HPLC on chiral stationary phase. b 50 °C and THF as solvent. c 220 mol% 1a , DQ, K 3 PO 4 and 100 mol% diol were used. Full size image Synthetic transformations In synthetic applications, our approach could be readily scaled up to 1.2 grams only with little influence on product yield (e.g., 3a , 1.2 grams, 79% yield, and >99:1 er; Fig. 2 ). The remaining aldehyde unit in our sulfoxide product 3a could be easily converted to a diverse set of functional groups (Fig. 3a ). For instance, the hydrogen of aldehyde could be deuterated [61] catalyzed by achiral NHC in the presence of D 2 O to afford 100% deuterated 4a in 77% yield and without the loss of optical purity. Moreover, the formyl group could be cyanation [62] and thioesterification catalyzed by achiral NHC with high er values ( 4b , 4c ). Enantioenriched terminal alkyne 4d and alkene 4e were synthesized efficiently by means of Seyferth–Gilbert reaction [63] and Wittig reaction [64] , respectively. Chiral sulfoxide 3a reacted with L–valinol [65] generated oxazolines 4 g was very similar to the SOX type ligands [66] , [67] (Fig. 1e ). Noteworthily, the chiral sulfoxide 4 h and its analogues have been proven as a chiral ligand and catalyst in several asymmetric synthesis [59] . It could be easily synthesized from 3a via reductive amination reaction as well as its analogues. Furthermore, 3a underwent hydrolysis of the ester group and subsequent reductive amination of the formyl group with BnNH 2 to afford an unnatural amino acid 4i bearing a chiral sulfoxide center with good yield and excellent er value. Combination of 3a with Ellman auxiliary [68] accessed to a chiral disulfoxide product 4j efficiently via a concise condensation reaction with 90% yield. Fig. 3: Synthetic transformations and applications. a K 3 PO 4 , NBS, 4 Å MS, 30 °C, toluene; b MgSO 4 , 4 h, CH 2 Cl 2 , NaBH 3 CN; c NaBH 4 , Ti(OEt) 4 , CH 2 Cl 2 ; d LiOH, THF:H 2 O = 2:1, 2 h, then 1 M HCl; e MgSO 4 , BnNH 2 , 4 h, then NaBH 3 CN; f Pyrrolidine, 4 Å MS, CH 2 Cl 2 , 60 °C; g achiral NHC, AcOK, D 2 O:CH 2 Cl 2 = 4:1; h achiral NHC, TsNH 2 , Et 2 NH, 4 Å MS, toluene; i achiral NHC, DQ, EtSH, K 3 PO 4 , CH 2 Cl 2 ; j TMSCHN 2 , LDA, THF, −78 °C; k CH 3 PPh 3 Br, KHMDS, THF; l Pd/C, H 2 , EtOH. a Synthetic transformation of 3 a . b Synthetic applications. Full size image Moreover, two practical applications of 4d and 4 g were verified. Alkyne 4d could be conjugated with an anti–HIV drug (Zidovudine) [69] which possessing an azido group to afford a modified Zidovudine 5a with moderate yield. As we expected, 4 g could be a potential chiral ligand in asymmetric synthetic chemistry, which was used as a chiral ligand in the Pd-catalyzed enantioselective substitution reaction [70] between the alkene 6 and the malonate 7 , with the chiral product 8 afforded in 98:2 er. (Fig. 3b ) Mechanistic studies To understand the possible impacts of chalcogen bonding interactions, we examined two other sulfoxide substrates ( 1aa and 1ab ) by placing the positions of aldehyde moieties which are far away from the sulfoxides sulfur center (Fig. 4a ). From analysis on the X–ray structure of 1aa , the remote aldehyde unit does not show any chalcogen bondind interaction with the sulfur atom (see Supplementary Table 2 ). It is therefore expected that the chalcogen bond–guided conformational resolution strategy developed here shall not work for substrates such as 1aa and 1ab . This expectation was verified by our experimental observations when the use of 1aa and 1ab under our condition, It gave the corresponding products ( 3aa and 3ac ) with nearly no enantiomeric excesses and the yields of di-esters were increased. Fig. 4: Mechanistic studies. a Control experiments without chalcogen bonding interaction. b Quantify the strength of chalcogen bonding interaction via DFT calculations. c Addition barrier of NHC to aldehyde moieties. d Oxidized barrier of Breslow intermediates. Full size image To probe further mechansic insights of our reactions, we investigated the chalcogen bonding strength between the sulfoxide and formyl group by using DFT calcuations (Fig. 4b ). The structure provided by single crystal diffraction data of 1a was used as the initial point for geometric optimizations. The chalcogen bond energy (ChBE) was estimated to be 3.44 kcal/mol (Fig. 4b ). Furthemore, in order to evalued the influence of substituents to the ChBs, substrates 1c (with OMe) and 1i (with CF 3 ) were examined with the same DFT calculation method. The initial structures for DFT calculations were obtained from the corresponding single crystall of 1c (CCDC 2172904 ) and 1i (CCDC 2172911 ). The results showed that the chalcogen bond strength of 1c and 1i were 3.56 and 4.27 kcal/mol, respectively (see Supplementary Fig. 1 for details). Moreover, the additions of NHC catalyst to aldehyde moiety in the two conformational isomers (two set of enantiomers; four possibilities for the additions) were then evaluated (Fig. 4c ). We found that the aldheyde moieties involved in chalcogen bonding interactions are conformationally locked and weakly activated. These conformationally locked aldehyde moieties react faster with the NHC catalsyt (ΔG ‡ = 5.50, 3.53 kcal/mol) than the no chalcogen bonded aldehyde moieties (ΔG ‡ = 6.49, 9.24 kcal/mol). Meantime, the low rotation barriers (Fig. 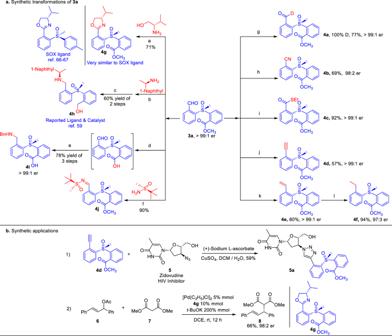Fig. 3: Synthetic transformations and applications. aK3PO4, NBS, 4 Å MS, 30 °C, toluene;bMgSO4, 4 h, CH2Cl2, NaBH3CN;cNaBH4, Ti(OEt)4, CH2Cl2;dLiOH, THF:H2O = 2:1, 2 h, then 1 M HCl;eMgSO4, BnNH2, 4 h, then NaBH3CN;fPyrrolidine, 4 Å MS, CH2Cl2, 60 °C;gachiral NHC, AcOK, D2O:CH2Cl2= 4:1;hachiral NHC, TsNH2, Et2NH, 4 Å MS, toluene;iachiral NHC, DQ, EtSH, K3PO4, CH2Cl2;jTMSCHN2, LDA, THF, −78 °C;kCH3PPh3Br, KHMDS, THF;lPd/C, H2, EtOH.aSynthetic transformation of 3a.bSynthetic applications. 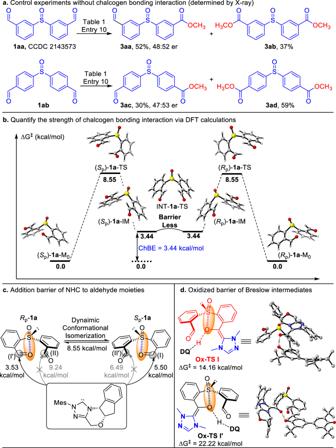Fig. 4: Mechanistic studies. aControl experiments without chalcogen bonding interaction.bQuantify the strength of chalcogen bonding interaction via DFT calculations.cAddition barrier of NHC to aldehyde moieties.dOxidized barrier of Breslow intermediates. 4b ) indicates that the conformations of 1a can undergo rapid interconversions at room temperature, making it feasible to achieve a carbene–catalyzed DKR process. Further DFT studies suggest that oxidation of the Breslow intermediate (Fig. 4d ) is the stereo–determine step. The activation energy difference of Ox–Ts I and Ox–Ts I′ (ΔG ‡ = 14.16, 22.22 kcal/mol, respectively) is estimated as 8.06 kcal/mol, suggesting an er value over 99:1, that is consistent with our experimental observations (see Supplementary Fig. 3 for details). In summary, we have disclosed a carbene-catalyzed DKR strategy for the synthesis of chiral sulfoxides. This method takes advantage of intramolecular chalcogen bonds installed in molecules to guide conformational isomerization and reactivity differentiation of substrates. In particular, through a chalcogen bonding–enabled reactivity differentiation, we realize a carbene–catalyzed dynamic kinetic resolution process for efficient preparation of chiral sulfoxides with excellent optical purities. The chiral sulfoxide products from our reactions may serve as platform scaffolds for straightforward transformation to useful molecules with applications in catalysis and biological studies. Chalcogen bonding interactions are naturally present or can be readily installed in various molecules. The strategy reported herein may open a new avenue in reaction control and asymmetric synthesis. General procedure for the catalytic reactions To a 100.0 mL over–dried round bottom flask equipped with a magnetic stir bar was added 1a (1.0 g, 3.87 mmol), DQ (1.58 g, 3.87 mmol), pre–NHC B (139.8 mg, 0.38 mmol) and K 3 PO 4 (164.2 mg, 0.77 mmol). The flask was then sealed, purged and backfilled with N 2 three times in glovebox before adding CH 2 Cl 2 (60.0 mL) and CH 3 OH (0.19 mL, 4.65 mmol), and the reaction mixture was stirred in oil bath at 30 °C for 12 h. The mixture was concentrated under reduced pressure. The resulting crude residue was purified via column chromatography on silica gel by using petroleum ether / ethyl acetate (2:1) to afford the desired product 3a (881.8 mg, 79% yield, > 99:1 er).